Learning-induced and stathmin-dependent changes in microtubule stability are critical for memory and disrupted in ageing Changes in the stability of microtubules regulate many biological processes, but their role in memory remains unclear. Here we show that learning causes biphasic changes in the microtubule-associated network in the hippocampus. In the early phase, stathmin is dephosphorylated, enhancing its microtubule-destabilizing activity by promoting stathmin-tubulin binding, whereas in the late phase these processes are reversed leading to an increase in microtubule/KIF5-mediated localization of the GluA2 subunit of AMPA receptors at synaptic sites. A microtubule stabilizer paclitaxel decreases or increases memory when applied at the early or late phases, respectively. Stathmin mutations disrupt changes in microtubule stability, GluA2 localization, synaptic plasticity and memory. Aged wild-type mice show impairments in stathmin levels, changes in microtubule stability and GluA2 localization. Blocking GluA2 endocytosis rescues memory deficits in stathmin mutant and aged wild-type mice. These findings demonstrate a role for microtubules in memory in young adult and aged individuals. In the brain, following neuronal activity there is an increase in synaptic transport, which results in the strengthening of synaptic connections, and ultimately in memory formation [1] . Among the many mechanisms mediating synaptic transport, cytoskeletal structures—actin filaments and microtubules—play a major role in motor-driven import and export [2] . Actin filaments are known to be dynamic and present in dendritic spines, where they play an essential role in synaptic function and memory formation [3] . Microtubule dynamics have been described in cell division, axonal pathfinding during development and axonal growth and regeneration. In contrast, in mature neurons, microtubules are generally viewed as stable non-dynamic structures present in dendritic shafts but not in dendritic spines. Intriguingly, recent work in hippocampal primary neuronal cultures indicates that microtubules can also be dynamically regulated during neuronal activity by moving from the dendritic shaft to the dendritic spines and affecting synaptic structure and function [4] , [5] , [6] , [7] , [8] , [9] . Despite this new information, the role of changes in microtubule stability in memory formation remains unclear. Microtubule assembly from heterodimers of α- and β-tubulins involves interaction with microtubule-associated proteins. One of these proteins, stathmin, binds tubulin heterodimers and prevents microtubule assembly, thus controlling microtubule dynamics [10] , [11] . When phosphorylated, stathmin releases tubulin dimers allowing microtubules to be formed [12] , [13] . Stathmin has been linked to fear, cognition and aging in rodent and human studies [14] , [15] , [16] , [17] , [18] , [19] , suggesting the involvement of microtubule dynamics in memory. Therefore, we set out to examine the role of stathmin-regulated control of microtubule stability in memory formation by focusing on learning-induced changes, because activity-dependent signalling is a hallmark of neuronal function [20] , [21] . Our approach reveals that by regulating microtubule stability and dendritic transport of the GluA2 subunit of AMPA-type glutamate receptors (AMPARs), stathmin controls synaptic plasticity and memory consolidation. Furthermore, we observe that aged wild-type (WT) mice, in addition to memory deficits, display deficits in stathmin levels, learning-dependent changes in microtubule stability and GluA2 dendritic transport along microtubules. Our combined approach demonstrates that learning-induced and stathmin-mediated changes in microtubule stability control GluA2 dendritic transport, synaptic plasticity and memory formation, pointing to a new learning-dependent intracellular signalling pathway. Stathmin activity is regulated by learning We first examined expression of stathmin protein in adult mice and found it to be present in the brain and testis ( Supplementary Fig. 1a ). In the brain, stathmin is located in the hippocampus, prefrontal cortex, amygdala, striatum, hypothalamus and cerebellum ( Supplementary Fig. 1b ). Stathmin is strongly expressed in the dentate gyrus with lesser expression in the CA3 and CA1 ( Supplementary Fig. 1c ). In the dentate gyrus, stathmin was found not only in the whole-cell extracts but also in the synaptosomal fraction ( Supplementary Fig. 1d ). Based on this observation, we focused our work on the dentate gyrus synaptosomes. To examine whether stathmin phosphorylation is regulated by learning, synaptosomal fractions from the dentate gyrus were isolated at several time points (5, 15 and 30 min, and 1, 2, 8 or 24 h) from mice subjected to single-shock contextual fear conditioning. Compared with naive mice, phosphorylation of synaptosomal stathmin at Ser16, Ser25 and Ser38 was rapidly decreased in mice 15–60 min following fear-conditioning training, and then phosphorylation of synaptosomal stathmin at Ser16 and Ser38 was increased 8 h following fear-conditioning training ( Fig. 1a and Supplementary Fig. 2 ). To confirm that the observed changes were specific to associative learning, we examined the effects of exposure to the context only (no shock) or the immediate shock deficit on stathmin phosphorylation ( Supplementary Fig. 3 ). In mice exposed to context only or to the immediate shock, phosphorylation of stathmin at Ser25 and Ser38 was rapidly decreased 30–60 min following the exposure, but no changes in phospho-stathmin levels were observed at 8 h. In contrast, there was no effect of either the context only or the immediate shock on stathmin phosphorylation at Ser16. 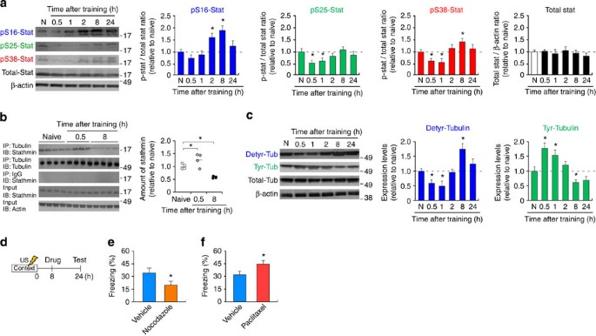Figure 1: Learning induces biphasic changes in stathmin activity and microtubule stability. (a) Immunoblot estimation of stathmin phosphorylation at Ser16 (pS16), Ser25 (pS25) and Ser38 (pS38), 0.5, 1, 2, 8 or 24 h following contextual fear conditioning. N, naive.n=6 per group (pooled tissues from three to four mice per sample). *P<0.05 versus naive mice (post-hoccomparison). (b) Analysis of stathmin-tubulin protein interactions using co-immunoprecipitation. Stathmin–tubulin complexes are formed at 0.5 h and dissociate at 8 h after contextual fear conditioning.n=4 per group (pooled tissues from four to five mice per sample). *P<0.05 (post-hoccomparison). (c) Immunoblot estimation of detyrosinated (Detyr-) and tyrosinated (Tyr-) α-tubulin levels after contextual fear conditioning.n=6 per group (pooled tissues from three to four mice per sample). *P<0.05 versus naive mice (post-hoccomparison). (d) Experimental design for drug administration 8 h following contextual fear conditioning. Memory was tested 24 h after training. (e) Mice injected with nocodazole 8 h following training show reduced freezing. vehicle,n=11; nocodazole,n=12. *P<0.05 (Student’st-test). (f) Mice injected with paclitaxel 8 h following training show increased freezing. vehicle,n=11; paclitaxel,n=12. *P<0.05 (Student’st-test). Data are expressed as mean±s.e.m. Figure 1: Learning induces biphasic changes in stathmin activity and microtubule stability. ( a ) Immunoblot estimation of stathmin phosphorylation at Ser16 (pS16), Ser25 (pS25) and Ser38 (pS38), 0.5, 1, 2, 8 or 24 h following contextual fear conditioning. N, naive. n =6 per group (pooled tissues from three to four mice per sample). * P <0.05 versus naive mice ( post-hoc comparison). ( b ) Analysis of stathmin-tubulin protein interactions using co-immunoprecipitation. Stathmin–tubulin complexes are formed at 0.5 h and dissociate at 8 h after contextual fear conditioning. n =4 per group (pooled tissues from four to five mice per sample). * P <0.05 ( post-hoc comparison). ( c ) Immunoblot estimation of detyrosinated (Detyr-) and tyrosinated (Tyr-) α-tubulin levels after contextual fear conditioning. n =6 per group (pooled tissues from three to four mice per sample). * P <0.05 versus naive mice ( post-hoc comparison). ( d ) Experimental design for drug administration 8 h following contextual fear conditioning. Memory was tested 24 h after training. ( e ) Mice injected with nocodazole 8 h following training show reduced freezing. vehicle, n =11; nocodazole, n =12. * P <0.05 (Student’s t -test). ( f ) Mice injected with paclitaxel 8 h following training show increased freezing. vehicle, n =11; paclitaxel, n =12. * P <0.05 (Student’s t -test). Data are expressed as mean±s.e.m. Full size image We examined whether the changes in stathmin phosphorylation following learning regulate stathmin–tubulin binding, which in turn may affect microtubule stability. Using co-immunoprecipitation on the synaptosomal fractions of the dentate gyrus, we found that stathmin binding to α-tubulin, a major component of microtubules, increased in the first 30 min but decreased the following 8 h after training ( Fig. 1b ). In mice exposed to context only, stathmin binding to α-tubulin was increased 30 min, but not 8 h, following the exposure ( Supplementary Fig. 4 ). These data suggest that during associative learning, stathmin may regulate microtubule stability by changing it’s affinity to α-tubulin. Changes in microtubule stability following learning To examine microtubule stability following learning, we measured the levels of the detyrosinated tubulin, a marker of stable microtubules, and tyrosinated tubulin, a marker of labile microtubules [22] , [23] , [24] . We found biphasic changes in tyrosinated and detyrosinated tubulin in the synaptosomal fractions of the dentate gyrus: detyrosinated tubulin levels were decreased 30–60 min and increased 8 h following contextual fear conditioning, whereas tyrosinated tubulin levels were changed in the opposite direction ( Fig. 1c and Supplementary Fig. 5 ). Similar to the changes in stathmin phosphorylation, exposure to context only ( Supplementary Fig. 6a ) or immediate shock ( Supplementary Fig. 6b ) led to a reduction of the detyrosinated tubulin and an increase in tyrosinated tubulin 0.5 h, but not 8 h, following the exposure. These results suggest that the increase in microtubule stability at 8 h is specific to associative learning. These results further suggest that microtubules become unstable 0.5–1 h and hyperstable 8 h following learning, and the increase in phospho-stathmin and subsequent microtubule hyperstability may be involved in memory consolidation. Memory can be enhanced by increasing microtubule stability We investigated whether pharmacological manipulation of the increase in microtubule stability following learning affects memory. We used paclitaxel or nocodazole to stabilize or destabilize microtubules, respectively. The drugs were injected into the dentate gyrus area of WT mice 8 h following fear conditioning, and memory was tested 24 h after training ( Fig. 1d ). Nocodazole injections decreased ( Fig. 1e ), while paclitaxel injections increased memory ( Fig. 1f ). To rule out the possibility that nocodazole injections disrupted freezing in a non-associative manner, we injected nocodazole into the dentate gyrus area of WT mice in home cage 24 h after they were subjected to contextual fear conditioning ( Supplementary Fig. 7 ). Their freezing responses were measured 48 h after training. There were no differences in freezing between mice injected with nocodazole and vehicle, thus suggesting that the nocodazole treatment alone did not disrupt freezing. These pharmacological experiments demonstrate that memory can be enhanced or disrupted by changing microtubule hyperstability 8 h following learning, and it also suggests that during this time period microtubule-dependent intracellular processes involved in memory consolidation are sensitive to manipulation. Stathmin controls microtubule stability and LTP To examine how stathmin-dependent microtubule stability may affect synaptic plasticity and memory, we employed transgenic mice expressing a mutant form of stathmin. Stathmin4A double-mutant mice ( Stat4A ) were generated using the tTA/tetO inducible bitransgenic system, which allows the Stathmin4A transgene to be turned on and off ( Fig. 2a ). The unphosphorylatable Stathmin4A gain-of-function mutant has its four Ser residue phosphorylation sites changed to Ala. Thus, it irreversibly binds α-tubulin, depleting cellular levels of free tubulin, and thus competing with endogenous stathmin and destabilizing microtubules [25] . Experimental mice were generated by crossing the GRP tTA knock-in mouse and tetO-Stat4A:GFP transgenic mouse. In the tetO-Stat4A:GFP transgenic line, Stathmin4A is fused to GFP under the control of the tTA-dependent tetO transcriptional operator. The Stat4A:GFP transgene is transcribed in the presence of tTA when these transgenic mice are crossed with the tTA-expressing line, GRP tTA knock-in mouse. Immunohistochemistry and western blotting revealed that the transgene was expressed in several brain areas, including the hippocampus, medial prefrontal cortex, anterior cingulate gyrus and amygdala ( Supplementary Fig. 8a,b ). Within the hippocampus, the Stat4A:GFP transgene was strongly expressed in the dentate gyrus ( Fig. 2b ) where it was present in neurons but not astrocytes ( Supplementary Fig. 8c ). The expression of the transgene did not affect the gross anatomy of the brain and the cilia in Stat4A mice ( Supplementary Fig. 8d,e ). The Stat4A:GFP transgene was expressed in the absence of the drug doxycycline ( Fig. 2c ; Off dox), but the transgene was turned off within 3 weeks after the dox was added to the diet (On dox). 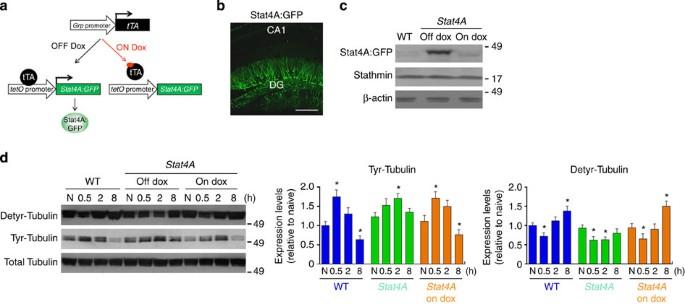Figure 2: Stathmin phosphorylation is essential for learning-dependent changes in microtubule stability. (a) Diagram illustrating transgenic design and control of transgene expression by doxycycline (dox) inStat4Abitransgenic mice. (b) Immunohistochemistry shows that Stat4A:GFP is expressed in the DG, but not CA1 area of the hippocampus. Scale bar, 200 μm. (c) Immunoblot using anti-GFP antibody demonstrates that transgene expression is repressed by dox. (d) Western blottings from the synaptosomal fraction of the DG ofStat4Amice show a deficit in microtubule hyperstability at 8 h after contextual fear conditioning. Tyr, tyrosinated tubulin; Detyr, detyrosinated tubulin. N, naive.n=6 per group (pooled tissues from three to four mice per sample). *P<0.05 versus naive in corresponding genotype (post-hoccomparison). Data are expressed as mean±s.e.m. Figure 2: Stathmin phosphorylation is essential for learning-dependent changes in microtubule stability. ( a ) Diagram illustrating transgenic design and control of transgene expression by doxycycline (dox) in Stat4A bitransgenic mice. ( b ) Immunohistochemistry shows that Stat4A:GFP is expressed in the DG, but not CA1 area of the hippocampus. Scale bar, 200 μm. ( c ) Immunoblot using anti-GFP antibody demonstrates that transgene expression is repressed by dox. ( d ) Western blottings from the synaptosomal fraction of the DG of Stat4A mice show a deficit in microtubule hyperstability at 8 h after contextual fear conditioning. Tyr, tyrosinated tubulin; Detyr, detyrosinated tubulin. N, naive. n =6 per group (pooled tissues from three to four mice per sample). * P <0.05 versus naive in corresponding genotype ( post-hoc comparison). Data are expressed as mean±s.e.m. Full size image We analysed microtubule stability in the dentate gyrus synaptosomal fraction of Stat4A mice following contextual fear conditioning. Western blotting revealed that detyrosinated tubulin levels were decreased 30 min after training in both Stat4A and WT mice, but Stat4A mice did not show an increase in detyrosinated tubulin levels at an 8-h time point, thus suggesting improper regulation of microtubule stability ( Fig. 2d ). Feeding Stat4A mice with dox for 3 weeks rescued the deficit ( Fig. 2d ). These results indicate that phosphorylation of stathmin is essential for microtubule hyperstability following learning. We tested synaptic strength and plasticity in Stat4A mice. Transgenic mice showed a trend to decrease maximum synaptic responses to afferent stimuli in the perforant path-dentate gyrus synaptic input ( Fig. 3a ), and a deficient θ -burst-induced long-term potentiation (LTP) ( Fig. 3b ). In contrast, synaptic strength and LTP at Schaffer collateral-CA1 synapses were normal ( Fig. 3c,d ). These experiments demonstrate that stathmin-dependent microtubule dynamics are critical for synaptic plasticity in the dentate gyrus. 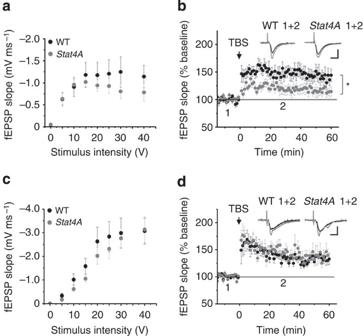Figure 3: Stathmin phosphorylation is essential for synaptic plasticity. (a) Input–output relationship of perforant path to dentate gyrus synaptic responses from WT and mutant mice (n=4, 6 slices). (b) Deficient perforant path to dentate gyrus LTP inStat4Amice (n=4, 6 slices). (c) Input–output relationship of Schaffer Collateral to CA1 (SC-CA1) synaptic responses from WT andStat4Amice. No effect is found on the relationship between stimulus strength and the size of postsynaptic response (input–output relationship). (d)Stat4Amice show normal LTP at SC-CA1 synapses. Averaged field EPSP data (n=4, 5 slices). *P<0.05 versus WT mice. Data are expressed as mean±s.e.m. Figure 3: Stathmin phosphorylation is essential for synaptic plasticity. ( a ) Input–output relationship of perforant path to dentate gyrus synaptic responses from WT and mutant mice ( n =4, 6 slices). ( b ) Deficient perforant path to dentate gyrus LTP in Stat4A mice ( n =4, 6 slices). ( c ) Input–output relationship of Schaffer Collateral to CA1 (SC-CA1) synaptic responses from WT and Stat4A mice. No effect is found on the relationship between stimulus strength and the size of postsynaptic response (input–output relationship). ( d ) Stat4A mice show normal LTP at SC-CA1 synapses. Averaged field EPSP data ( n =4, 5 slices). * P <0.05 versus WT mice. Data are expressed as mean±s.e.m. Full size image Context fear memory is dependent on dentate gyrus stathmin Next, we examined how the deficiency in microtubule hyperstabilization at the 8-h time point might affect memory in Stat4A mice. In single-shock contextual fear conditioning, Stat4A mice showed a deficit in long-term memory (24 h), which was rescued by dox at the adult stage ( Fig. 4a ). In contrast, there was no significant difference in short-term memory (0.5 h) in Stat4A mice ( Fig. 4b ). Stat4A mice were normal in tone-shock single pairing cued fear conditioning ( Fig. 4c ), which is dependent on the amygdala but not on the hippocampus. We also examined the role of stathmin in spatial memory using the Morris water maze and Barnes maze. In the Morris water maze test, Stat4A mice showed a deficit in initial spatial learning and reversed learning but were normal in the probe test ( Fig. 4d–g ). In the Barnes maze, we found that the spatial coordinates of the target box was delayed for Stat4A mice compared with WT control animals ( Fig. 4h ). The results from these two independent memory paradigms confirm impairment in hippocampus-dependent memory in Stat4A mice. 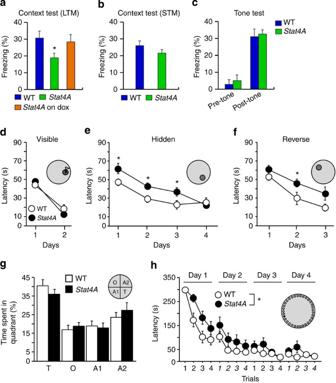Figure 4: Stathmin phosphorylation is essential for hippocampus-dependent memory. (a) Deficient long-term (24 h) contextual fear memory inStat4Amice is rescued by dox. WT,n=14;Stat4A,n=15;Stat4Aon dox,n=14. *P<0.05 versus WT mice (post-hoccomparison). (b) Normal short-term (0.5 h) memory inStat4Amice.n=10 per group. (c) Cued fear memory is normal inStat4Amice.n=14 per group. (d–g) Morris water maze. There was no difference in the visible platform task between the genotypes (d). In hidden platform, the latencies ofStat4Amice were slower than those of WT mice (e). In the reversal learning (transfer task),Stat4Amice showed longer latency to find the platform (f). The probe trial (g) shows normal spatial memory recall inStat4Amice.n=10 for each group. *P<0.05. (h) Reduced spatial learning inStat4Amice assessed in Barnes maze.n=11 for each group. *P<0.05. Data are expressed as mean±s.e.m. Figure 4: Stathmin phosphorylation is essential for hippocampus-dependent memory. ( a ) Deficient long-term (24 h) contextual fear memory in Stat4A mice is rescued by dox. WT, n =14; Stat4A , n =15; Stat4A on dox, n =14. * P <0.05 versus WT mice ( post-hoc comparison). ( b ) Normal short-term (0.5 h) memory in Stat4A mice. n =10 per group. ( c ) Cued fear memory is normal in Stat4A mice. n =14 per group. ( d – g ) Morris water maze. There was no difference in the visible platform task between the genotypes ( d ). In hidden platform, the latencies of Stat4A mice were slower than those of WT mice ( e ). In the reversal learning (transfer task), Stat4A mice showed longer latency to find the platform ( f ). The probe trial ( g ) shows normal spatial memory recall in Stat4A mice. n =10 for each group. * P <0.05. ( h ) Reduced spatial learning in Stat4A mice assessed in Barnes maze. n =11 for each group. * P <0.05. Data are expressed as mean±s.e.m. Full size image Anxiety tested in the open field and elevated plus maze was normal ( Supplementary Fig. 9a–c ) in Stat4A mice. In addition, depression-like behaviours assessed by the forced swim test and sucrose preference tests were normal in Stat4A mice ( Supplementary Fig. 9d,e ). Thus, deficits in stathmin-dependent microtubule stability lead to a decrease in contextual fear memory without affecting cued fear memory, anxiety or depression-like behaviour in Stat4A mice. Stat4A mice express the transgene in the dentate gyrus area and have a deficiency in perforant path-dentate gyrus LTP but have a normal Schaffer collateral-CA1 LTP, suggesting that improper dentate gyrus microtubule function may be responsible for the deficits in contextual fear memory. However, transgene expression in the amygdala and some cortical areas may also affect contextual fear conditioning in these mice. To confirm that the deficits in contextual fear conditioning are caused by changes in dentate gyrus microtubules, we overexpressed the Stathmin4A transgene in the dentate gyrus of WT mice using adeno-associated virus (AAV)-mediated gene transfer ( Fig. 5a ). The levels of the detyrosinated tubulin in mice injected with AAV-Stat4A-IRES-GFP in the dentate gyrus were normal 30 min, but decreased 8 h following learning ( Fig. 5b,c ). These mice also displayed reduced contextual fear memory compared with control mice injected with AAV-GFP ( Fig. 5d ). These results show that learning-induced and stathmin-dependent changes in microtubule stability in the dentate gyrus are critical for contextual fear memory. 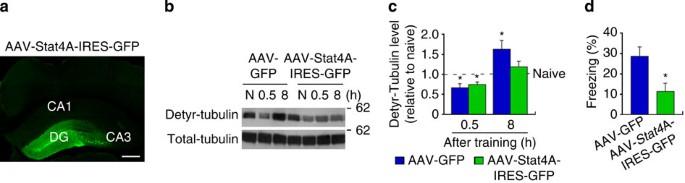Figure 5: Stathmin control of microtubule stability in the dentate gyrus is critical for contextual fear conditioning. (a) AAV-mediated overexpression ofStat4Ain the dentate gyrus (DG) detected by immunohistochemistry with anti-GFP antibody. Scale bar, 200 μm. (b,c) Immunoblot estimation of detyrosinated α-tubulin levels 0.5 h after training in the DG synaptosomal fraction of mice injected withAAV-GFPorAAV-Stat4A-IRES-GFP.N, naive.n=5–7 per group (pooled tissues from three to four mice per sample). *P<0.05 versus naive mice (Student’st-test). (d) AAV-mediated overexpression ofStat4Areduces contextual fear memory.n=11–12 per group. *P<0.01 (Student’st-test). Data are expressed as mean±s.e.m. Figure 5: Stathmin control of microtubule stability in the dentate gyrus is critical for contextual fear conditioning. ( a ) AAV-mediated overexpression of Stat4A in the dentate gyrus (DG) detected by immunohistochemistry with anti-GFP antibody. Scale bar, 200 μm. ( b , c ) Immunoblot estimation of detyrosinated α-tubulin levels 0.5 h after training in the DG synaptosomal fraction of mice injected with AAV-GFP or AAV-Stat4A-IRES-GFP. N, naive. n =5–7 per group (pooled tissues from three to four mice per sample). * P <0.05 versus naive mice (Student’s t- test). ( d ) AAV-mediated overexpression of Stat4A reduces contextual fear memory. n= 11–12 per group. * P <0.01 (Student’s t -test). Data are expressed as mean±s.e.m. Full size image Role of learning-induced microtubule instability in memory Next, we investigated microtubule instability occurring 0.5 h after learning using paclitaxel injections in the dentate gyrus area of WT mice. As the level of the detyrosinated tubulin in WT mice was decreased 0.5–1 h following learning ( Fig. 1c ), we injected paclitaxel immediately after contextual fear conditioning to inhibit microtubule destabilization. Memory was assessed 24 h following training ( Fig. 6a ). We found that mice injected with paclitaxel had reduced contextual fear memory. 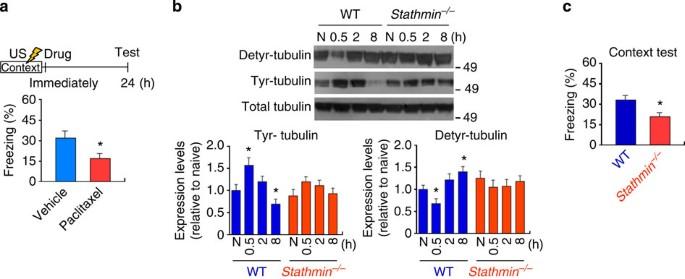Figure 6: Role of learning-induced microtubule instability in memory. (a) Mice injected with paclitaxel immediately following training show reduced freezing. Vehicle,n=11; Paclitaxel,n=12. *P<0.05 (Student’st-test). (b) stathmin−/−mice show deficit in microtubule destability and stability at 0.5 and 8 h after training.n=6 per group (pooled tissues from three to four mice per sample). N, naive. *P<0.05 versus naive in corresponding genotype (post-hoccomparison). (c) stathmin−/−mice show reduced long-term (24 h) contextual fear memory.n=12 per group. *P<0.01 (Student’st-test). Figure 6: Role of learning-induced microtubule instability in memory. ( a ) Mice injected with paclitaxel immediately following training show reduced freezing. Vehicle, n =11; Paclitaxel, n =12. * P <0.05 (Student’s t -test). ( b ) s tathmin −/− mice show deficit in microtubule destability and stability at 0.5 and 8 h after training. n =6 per group (pooled tissues from three to four mice per sample). N, naive. * P <0.05 versus naive in corresponding genotype ( post-hoc comparison). ( c ) s tathmin −/− mice show reduced long-term (24 h) contextual fear memory. n =12 per group. * P <0.01 (Student’s t -test). Full size image We also investigated the effect of stathmin loss-of-function mutation on microtubule stability and memory using stathmin −/− mice. In contrast to WT mice, there were no changes in the detyrosinated and tyrosinated α-tubulin levels in the dentate gyrus synaptosomal fractions in stathmin −/− mice 30 min and 8 h following contextual fear conditioning ( Fig. 6b ). Stathmin −/− mice had normal gross brain morphology ( Supplementary Fig. 10 ) and were deficient in contextual fear memory tested 24 h after training ( Fig. 6c ). These data indicate that in the absence of stathmin, both early instability and late hyperstability in microtubules are deficient following learning, leading to deficits in memory formation. Stathmin regulates learning-dependent GluA2 localization Which downstream events are regulated by stathmin-dependent changes in microtubule stability? Microtubules in dendrites of mature neurons are mainly responsible for intracellular transport [2] . Learning-induced AMPA-type glutamate receptors are delivered to spines in the hippocampus, which are critical for synaptic plasticity [26] and contextual memory [27] , [28] . Principal neurons in the adult brain express AMPARs that predominately contain the GluA2 subunit [29] . Therefore, we injected AAV-Stat4A-IRES-GFP in the dentate gyrus to examine whether learning-induced intracellular transport of GluA2 along dendrites is regulated by stathmin-dependent changes in microtubule stability. The amount of GluA2 in the dentate gyrus synaptosomal fractions of WT mice injected with the control AAV-GFP virus significantly increased 8 h after contextual fear conditioning, whereas mice injected with the AAV-Stat4A-IRES-GFP did not show an increase in GluA2 ( Fig. 7a ). GluA2 levels were the same in the whole-cell extracts from mice injected with the AAV-GFP or AAV-Stat4A-IRES-GFP ( Fig. 7b ), suggesting that an increase in GluA2 levels in the synaptosomal fractions after learning might be caused by enhanced dendritic transport from the soma to the dendritic shaft along the hyperstable microtubules. Indeed, the GluA2 levels in the microtubule fractions were significantly increased after training in control mice injected with the AAV-GFP , whereas mice injected with AAV-Stat4A-IRES-GFP did not show increased GluA2 ( Fig. 7c ). 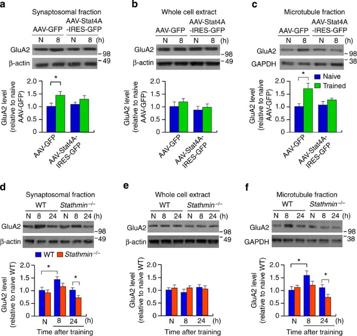Figure 7: Stathmin regulates learning-dependent dendritic transport of GluA2. (a–c) Immunoblot estimation of the level of GluA2 in synaptosomal (a,n=8 per group, pooled tissues from three to four mice per sample whole cell extract (b,n=4 per group) and microtubule (c,n=4 per group, pooled tissues from three to four mice per sample) fractions of the DG in mice injected withAAV-GFPorAAV-Stat4A-IRES-GFPin naive and 8 h after training conditions. *P<0.05 (post-hoccomparison). (d–f) Reduced GluA2 synaptic transport instathmin−/−mice, as analysed by immunoblotting, in the synaptosomal (d,n=4 per group, pooled tissues from three to four mice per sample), whole cell extract (e,n=4 per group) and microtubule (f,n=4 per group, pooled tissues from three to four mice per sample) fractions in naive and trained mice. *P<0.05 (post-hoccomparison). Data are expressed as mean±s.e.m. Figure 7: Stathmin regulates learning-dependent dendritic transport of GluA2. ( a – c ) Immunoblot estimation of the level of GluA2 in synaptosomal ( a , n =8 per group, pooled tissues from three to four mice per sample whole cell extract ( b , n =4 per group) and microtubule ( c , n =4 per group, pooled tissues from three to four mice per sample) fractions of the DG in mice injected with AAV-GFP or AAV-Stat4A-IRES-GFP in naive and 8 h after training conditions. * P <0.05 ( post-hoc comparison). ( d – f ) Reduced GluA2 synaptic transport in stathmin −/− mice, as analysed by immunoblotting, in the synaptosomal ( d , n =4 per group, pooled tissues from three to four mice per sample), whole cell extract ( e , n =4 per group) and microtubule ( f , n =4 per group, pooled tissues from three to four mice per sample) fractions in naive and trained mice. * P <0.05 ( post-hoc comparison). Data are expressed as mean±s.e.m. Full size image Next, we examined whether learning induces changes in the GluA2 levels in stathmin −/− mice. In contrast to WT mice, stathmin −/− mice did not show an increase in the GluA2 levels in the synaptosomal fractions at the 8-h time point ( Fig. 7d ). The GluA2 levels were normal in the whole-cell extracts in stathmin −/− mice ( Fig. 7e ). Similar to the synaptosomal fraction, the GluA2 levels in the microtubule fraction were not increased 8 h following training in stathmin −/− mice, whereas WT mice showed an increase in the GluA2 levels ( Fig. 7f ). These results suggest that learning promotes GluA2 localization to the synaptic sites in stathmin- and microtubule-dependent manner. To examine whether synaptic GluA2 levels are also altered by stathmin mutation, we investigated GluA2 localization by fractionation of synaptosomes. We performed further digestion of synaptosomes to yield an insoluble ‘postsynaptic density (PSD)-enriched’ membrane fraction and a ‘non-PSD enriched’ membrane fraction ( Supplementary Fig. 11 ) [30] , [31] . We found increased GluA2 in both the synaptic PSD and non-PSD fractions in WT mice 8 h after learning, whereas there was no difference in the GluA2 levels either in the PSD and non-PSD fractions from the WT mice injected with the AAV-Stat4A-IRES-GFP , as well as from stathmin −/− mice ( Supplementary Fig. 12 ). We also examined whether disruption of learning-induced microtubule hyperstability influences increase in synaptosomal and synaptic GluA2. WT mice were injected with nocodazole 2 h after contextual fear conditioning and were euthanized 8 h after training ( Supplementary Fig. 13a ). We found increased GluA2 levels in PSD and synaptosomal fractions, but not in whole-cell extracts, in vehicle-treated mice ( Supplementary Fig. 13b ). However, we did not find an enhancement of the GluA2 levels either in the PSD or synaptosomal fractions in nocodazole-treated mice ( Supplementary Fig. 13b ). These results further confirm that changes in microtubule stability following learning are critical for synaptosomal and synaptic localization of GluA2. Stathmin-dependent binding of KIF5 to microtubules and GluA2 We further investigated how stathmin regulates dendritic GluA2 localization following learning. Tubulin detyrosination (a marker of stable microtubules) induces kinesin motor protein KIF5 binding to microtubules as well as its motor activity [32] . Moreover, in dendrites, GluA2 is transported by KIF5 (ref. 33 ). This led us to speculate that learning-induced tubulin detyrosination activated both KIF5 binding to microtubules and KIF5-dependent GluA2 transport. We performed co-immunoprecipitation to examine the binding of GluA2 to KIF5, KIF5 to α-tubulin and GluA2 to α-tubulin in the hippocampus after contextual fear conditioning. After training, the binding of GluA2 to α-tubulin, KIF5 to α-tubulin and KIF5 to GluA2 was increased in WT mice but not in stathmin −/− mice ( Fig. 8a–c ), suggesting that KIF5 may be a molecular link that connects stathmin and microtubules to activity-dependent dendritic transport of GluA2. 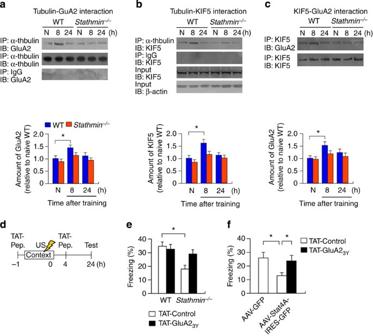Figure 8: Stathmin controls learning-induced dendritic transport of GluA2 by modulating binding of motor protein KIF5 to microtubules. Co-immunoprecipitation reveals deficiency in protein binding between GluA2 and α-tubulin (a), KIF5 and α-tubulin (b), and GluA2 and KIF5 (c) instathmin−/−mice. N, naive.n=4 per group (pooled tissues from two to three mice per sample). *P<0.05 (post-hoccomparison). (d) Scheme of the experimental design and TAT-GluA23Ypeptide (TAT-Pep.) injection schedule is shown. (e) Blocking GluA2 endocytosis by intra-hippocampal injection of TAT-GluA23Ypeptide has no effect in WT mice, but rescues contextual fear memory instathmin−/−mice.n=12–13. *P<0.05 versus mice given TAT-control peptide (post-hoc comparison). (f) Rescue of contextual fear memory by TAT-GluA23Ypeptide in WT mice injected withAAV-Stat4A-IRES-GFP.n=10–12. *P<0.05 (post-hoccomparison). Data are expressed as mean±s.e.m. Figure 8: Stathmin controls learning-induced dendritic transport of GluA2 by modulating binding of motor protein KIF5 to microtubules. Co-immunoprecipitation reveals deficiency in protein binding between GluA2 and α-tubulin ( a ), KIF5 and α-tubulin ( b ), and GluA2 and KIF5 ( c ) in stathmin −/− mice. N, naive. n =4 per group (pooled tissues from two to three mice per sample). * P <0.05 ( post-hoc comparison). ( d ) Scheme of the experimental design and TAT-GluA2 3Y peptide (TAT-Pep.) injection schedule is shown. ( e ) Blocking GluA2 endocytosis by intra-hippocampal injection of TAT-GluA2 3Y peptide has no effect in WT mice, but rescues contextual fear memory in stathmin −/− mice. n =12–13. * P <0.05 versus mice given TAT-control peptide ( post-ho c comparison). ( f ) Rescue of contextual fear memory by TAT-GluA2 3Y peptide in WT mice injected with AAV-Stat4A-IRES-GFP . n =10–12. * P <0.05 ( post-hoc comparison). Data are expressed as mean±s.e.m. Full size image Blocking GluA2 endocytosis rescues memory deficits To further examine the role of stathmin-mediated dendritic transport of GluA2, we decided to examine whether increasing the amount of GluA2 at the synapse would rescue contextual fear memory in stathmin −/− mice. A synthetic peptide TAT-GluA2 3Y , known to inhibit GluA2 endocytosis without decreasing basal synaptic transmission or LTP [34] , was injected in the dentate gyrus area. This peptide has an estimated half-life time 250–300 min after intravenous injection [34] . To increase the time of its action, we injected the peptide twice, 1 h before and 4 h after training ( Fig. 8d ). There was no significant difference in freezing between WT mice injected with either the TAT-GluA2 3Y or TAT-control peptides ( Fig. 8e ). However, freezing of stathmin −/− mice injected with the TAT-GluA2 3Y was significantly increased compared with stathmin −/− mice injected with the TAT-control peptide ( Fig. 8e ). We also examined whether the TAT-GluA2 3Y peptide had an effect on contextual fear memory in WT mice injected with AAV-Stat4A-IRES-GFP . The freezing response in mice injected with AAV-Stat4A-IRES-GFP and TAT-GluA2 3Y peptide was significantly increased compared with mice injected with AAV-Stat4A-IRES-GFP and TAT-control peptide ( Fig. 8f ). Thus, blocking GluA2 endocytosis rescued memory both in stathmin −/− mice and WT mice injected with AAV-Stat4A-IRES-GFP . This suggests that GluA2 synaptic localization in the dentate gyrus is at least partially mediated by stathmin-dependent microtubule dynamics, and this process is critical for contextual fear memory. Stathmin-microtubule connection to aged-related memory loss Previous work implicated stathmin in ageing in healthy humans [18] . Furthermore, the dentate gyrus is vulnerable to the effects of normal ageing in humans and primates [35] , [36] . Indeed, aged mice showed reduced contextual fear memory ( Fig. 9 ). We therefore examined stathmin-microtubule interactions in age-dependent memory loss. Intriguingly, similar to the work in humans, we found that stathmin expression in the dentate gyrus of the hippocampus gradually decreased from 2 to 12 to 18 months in naive WT mice ( Fig. 10a ). We analysed post-translational modifications of α-tubulin following contextual fear conditioning in the synaptosomal fractions of the dentate gyrus of 18-month-old mice. In contrast to young adult mice, aged mice showed a significant attenuation of changes in detyrosinated tubulin ( Fig. 10b ), suggesting improper regulation of microtubule stability. Next, we measured GluA2 levels in mice subjected to contextual fear conditioning with one or three foot shocks, and found a significant difference between young adult and aged mice. The GluA2 levels in the dentate gyrus synaptosomal and microtubule fractions were not increased in aged mice after training (one foot shock) ( Fig. 10c–e ). Furthermore, the aged mice needed a stronger stimulus to reach the levels of GluA2 found in the young adults. To confirm whether the deficit in synaptosomal GluA2 in trained aged mice causes memory deficits, we analysed contextual fear memory after injecting TAT-GluA2 3Y peptide into the dentate gyrus area of aged mice. We found that TAT-GluA2 3Y rescued fear memory of aged mice to the level of young adults that received the TAT-control peptide ( Fig. 10f ). Thus, stathmin-dependent microtubule stability is involved in both regulating memory consolidation in young adult mice and in age-associated memory loss, suggesting that stathmin–microtubule interactions represent a general mechanism for memory formation. 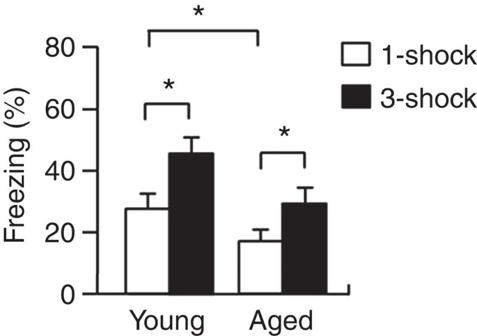Figure 9: Decreased contextual fear memory in aged WT mice. Aged (16–20 months old) and young adult (2–4 months old) WT mice were subjected to one-footshock or three-footshock contextual fear conditioning. Memory was tested 24 h following training. Aged mice showed reduced contextual fear memory.n=11–13 per group.P<0.05 (post-hoccomparison). Data are expressed as mean±s.e.m. Figure 9: Decreased contextual fear memory in aged WT mice. Aged (16–20 months old) and young adult (2–4 months old) WT mice were subjected to one-footshock or three-footshock contextual fear conditioning. Memory was tested 24 h following training. Aged mice showed reduced contextual fear memory. n =11–13 per group. P <0.05 ( post-hoc comparison). Data are expressed as mean±s.e.m. 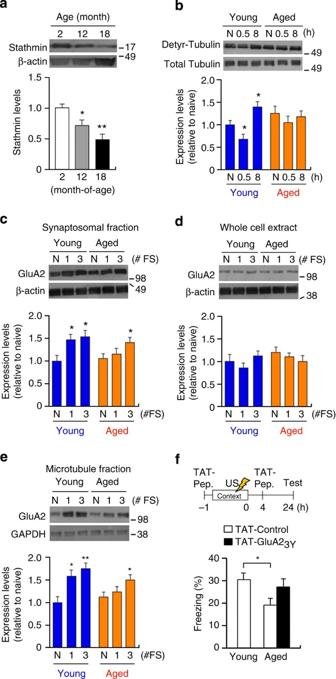Figure 10: Age-dependent memory loss is associated with microtubule-dependent dendritic transport of GluA2. (a) Immunoblotting shows reduced level of total stathmin protein in the dentate gyrus (DG) of aged WT mice.n=5 per group. *P<0.05, **P<0.01 versus young adult mice (post-hoccomparison). (b) Immunoblotting shows deficiency in learning-dependent microtubule destability and hyperstability in aged mice. Detyr, detyrosinated. N, naive.n=5 per group (pooled tissues from threeto four mice per sample). *P<0.05 versus naive young adult mice (post-hoccomparison). (c–e) Immunoblot estimation of GluA2 levels in aged mice in synaptosomal (c,n=5 per group, pooled tissues from three to four mice per sample), whole cell extract (d,n=5 per group) and microtubule (e,n=5 per group, pooled tissues from 3–4 mice per sample) fractions of the DG of naïve and trained (single or three foot-shock pairings) aged and young adult mice. N, naive; #FS, number of foot-shocks; 1, one foot shock; 3, three foot shocks. *P<0.05, **P<0.01 versus naive mice in corresponding group (post-hoccomparison). (f) Intra-hippocampal injection of the TAT-GluA23Ypeptide rescued decreased contextual fear memory in aged mice.n=12–13. *P<0.05 (post-hoccomparison). Data are expressed as mean±s.e.m. Full size image Figure 10: Age-dependent memory loss is associated with microtubule-dependent dendritic transport of GluA2. ( a ) Immunoblotting shows reduced level of total stathmin protein in the dentate gyrus (DG) of aged WT mice. n =5 per group. * P <0.05, ** P <0.01 versus young adult mice ( post-hoc comparison). ( b ) Immunoblotting shows deficiency in learning-dependent microtubule destability and hyperstability in aged mice. Detyr, detyrosinated. N, naive. n =5 per group (pooled tissues from threeto four mice per sample). * P <0.05 versus naive young adult mice ( post-hoc comparison). ( c – e ) Immunoblot estimation of GluA2 levels in aged mice in synaptosomal ( c , n =5 per group, pooled tissues from three to four mice per sample), whole cell extract ( d , n =5 per group) and microtubule ( e , n =5 per group, pooled tissues from 3–4 mice per sample) fractions of the DG of naïve and trained (single or three foot-shock pairings) aged and young adult mice. N, naive; #FS, number of foot-shocks; 1, one foot shock; 3, three foot shocks. * P <0.05, ** P <0.01 versus naive mice in corresponding group ( post-hoc comparison). ( f ) Intra-hippocampal injection of the TAT-GluA2 3Y peptide rescued decreased contextual fear memory in aged mice. n =12–13. * P <0.05 ( post-hoc comparison). Data are expressed as mean±s.e.m. Full size image Our work demonstrates that learning induces biphasic changes in stathmin phosphorylation, which trigger changes in stathmin-tubulin binding and microtubule stability, leading in turn to increases in GluA2 localization at the synaptic sites, promoting synaptic plasticity and long-term memory. On the other hand, perturbations of the stathmin’s function to control microtubule stability lead to deficits in GluA2 localization, synaptic plasticity and memory formation. We found a decrease and then a subsequent increase in stathmin phosphorylation 15 min–0.5 h (early phase) and 8 h following learning (late phase). Although phosphorylation of stathmin at all Ser residues is important for inactivation of its depolymerization activity [37] , [38] , phosphorylation at Ser16 strongly reduces the binding affinity of stathmin to tubulin heterodimers [12] , [13] , [39] . Ser16 can be phosphorylated by protein kinase A and calmodulin-dependent protein kinase II/IV [40] , [41] , [42] , the kinases critically involved in memory formation [43] , [44] , [45] . Thus, it is highly likely that the kinases and phosphatases controlling stathmin phosphorylation may have an important role in memory formation by controlling microtubule stability. We found two distinct phases of changes in microtubule stability: 0.5–1 h following learning when microtubules become unstable (early phase) and 8 h following learning when microtubules become hyperstable (late phase). These results are based on the measurements of microtubule stability using antibodies against tyrosinated and detyrosinated tubulin. Although these measurements assess microtubule stability indirectly, they have been used in a number of studies, including those when testing of stathmin-dependent microtubule stability in brain tissue was analysed [24] , [46] . Biphasic changes in stathmin-tubulin binding, similar to changes in stathmin phosphorylation, provide further support to the notion that microtubules change their stability. Importantly, local injections of a microtubule-stabilizing drug paclitaxel at the early phase disrupt, whereas injections at the late phase enhance, long-term memory. Microtubule hyperstability during the late phase appears to be specifically related to associative learning (context-unconditioned stimulus (US) presentation), because this change is not seen after exposure to context only or immediate shock. In contrast, the early-phase changes occur not only after context-US but also after exposure to context only or immediate shock. Thus, the early phase seems to be involved in attention/arousal/US-related events as well as associative memory. It is important to note that manipulating microtubule stability at the early phase also disrupts memory, suggesting that the early phase is necessary for memory formation. We speculate that during the early phase, initial microtubule disassembly caused by increased stathmin activity is likely to trigger subsequent assembly of new microtubules, which are then stabilized during the late phase, allowing an increase in dendritic transport. Our work in live animals suggests that stathmin-dependent changes in microtubule stability are involved in synaptic function and memory formation. The learning-dependent changes in microtubule stability we observed are in agreement with activity-dependent changes in microtubules found at the synapse in hippocampal primary cell cultures [4] , [5] , [6] , [7] , [8] , [9] . Although our data are supported by other literature, suggesting that microtubule function is important for memory formation [47] , [48] , [49] , its molecular mechanisms remain to be elucidated. Our data provide the mechanism of how learning-induced stathmin phosphorylation regulates microtubule stability and long-term memory formation. In particular, our work is in agreement with Fanara et al. [49] whose study implicates microtubule turnover in learning. A recent study has shown that the levels of stathmin mRNA and protein are increased 2 days following contextual fear conditioning [50] . It is possible that the increases in stathmin levels found in that paper reflect the compensational changes caused by the earlier use of stathmin on day one following learning as our work demonstrates. These findings are in agreement with our work showing that learning induces changes in stathmin in the dentate gyrus. We found the phospho-stathmin levels to be decreased 15 min and then increased 8 h following training; there were no differences in total stathmin levels at these time points. We also found the levels of total and phospho-stathmin to be normal 24 h following training. Although both studies used single-shock contextual fear conditioning, we still cannot exclude that the differences in the results may reflect the specific details of the training paradigms. We showed that stathmin-mediated control of microtubule stability regulates the binding properties of the GluA2-KIF5 motor protein complex and dendritic GluA2 localization. Our observations of enhanced tubulin detyrosination and increased interactions of KIF5 and α-tubulin occurring 8 h following learning are in agreement with the finding in the hippocampal primary cell cultures that tubulin detyrosination enhances the motor activity of KIF5 and its binding to microtubules [32] . We also found that KIF5-GluA2 interactions and synaptosomal and synaptic (PSD fractions) GluA2 levels were increased 8 h following learning. However, stathmin mutant mice have deficits in learning-induced GluA2-KIF5 interactions and synaptosomal and synaptic GluA2 localization. KIF5 is known to control intracellular transport of AMPARs [33] , and the insertion of AMPARs into spines during synaptic plasticity requires a myosin motor protein [26] , [51] . Given the fact that the GluA2 levels in the non-PSD fractions were also deficient in stathmin mutant mice, the deficiency in synaptic GluA2 localization in stathmin mutant mice might be caused by dysregulation of GluA2 transport from the soma to the dendritic shaft along microtubules. However, synaptic transport can also be deficient, as a recent study has shown that KIF5 regulates synaptic delivery and redistribution of AMPARs [52] . Although the molecular mechanisms of synaptic AMPARs delivery are still unclear, our data suggest that stathmin regulates dendritic transport of GluA2 by regulating microtubule stability during memory formation. The ability of the blocker of GluA2 endocytosis to rescue contextual fear memory in stathmin mutant mice is in agreement with the role of AMPAR transport in synaptic plasticity and contextual memory [26] , [27] , [28] , [53] , [54] , [55] . Therefore, GluA2 intracellular localization at the synaptosomes is controlled by changes in microtubule stability in a learning-dependent manner and these interactions serve as a molecular link to synaptic function and memory formation. Consistent with stronger expression of both the endogenous stathmin and Stathmin4A transgene in the dentate gyrus compared with other areas of the hippocampus, we found that perforant path-dentate gyrus LTP, but not Schaffer collateral-CA1 LTP, is deficient in Stat4A mice. Furthermore, WT mice expressing virus-mediated Stathmin4A in the dentate gyrus showed deficiency in contextual fear memory. Taken together, these results demonstrate an essential role of stathmin–microtubule interactions in dentate gyrus synaptic plasticity and contextual fear memory. The timing of the changes of stathmin phosphorylation that we observed in brain sections is different from the timing of LTP induction. One possibility is that learning in live animals and LTP induction in slices may be dependent on somewhat different molecular mechanisms. Other possibilities include changes in localization of certain synaptic molecules in naive condition that lead to a deficit in LTP induction in Stat4A mice. Although our data suggest that dysregulation of dendritic transport of GluA2 in stathmin mutant mice is observed only following learning, we cannot exclude the possibility that stathmin regulates dendritic localization of other molecules even in naive conditions. Some of the candidates may include kinesin motor proteins as well as their cargo [56] . How general is this signalling pathway for memory formation? To begin answering this question, we turned to ageing-associated memory loss focusing on the dentate gyrus, as it is implicated in normal ageing in humans and primates [35] , [36] . Interestingly, stathmin expression in the human brain is decreased with ageing [18] and this decrease is accelerated in Alzheimer’s disease [18] , [57] , [58] . We found that aged mice show decreased stathmin levels and lack of learning-induced increase in GluA2 levels in synaptosomal and microtubule fractions. Furthermore, blocking the GluA2 endocytosis reverses the deficits in contextual fear memory in aged mice, suggesting that the GluA2 dendritic transport has an important role in age-dependent memory loss. This is consistent with a recent report showing that reduced levels of the synaptic GluA2 in the dentate gyrus are associated with memory loss in aged monkeys [59] . In conclusion, our data demonstrate that learning-dependent regulation of GluA2 dendritic transport by stathmin-mediated changes in microtubule stability is crucial for memory formation and dysfunction in this signalling pathway might be one of the mechanisms underlying age-dependent memory loss. Thus, changing stathmin activity or microtubule stability might be a useful approach to regulate memory formation. Given that improving microtubule stability was proposed as an approach to establishing axonal and synaptic connections in spinal cord injury and central nervous system lesions [47] , [60] , [61] , controlling microtubule stability may be a convergent pathway for different biological processes of the nervous system. Animals Male C57BL/6J mice were purchased from Jackson Laboratory. Generation of the GRP tTA knock-in mice. The portion of the mouse Grp gene, 4.5 kb long, which includes exon 1 was isolated and the Not I– Asc I site inserted in front of the ATG in exon 1, generating a plasmid pGP109(NA). The humanized htTA gene (gift from Dusan Bartsch) was inserted into the plasmid pnCreFNF14.19 (after removing nCre complementary DNA; gift from Xiaoxi Zhuang), generating ptTAFNF. A plasmid pGP109-tTA-FNF was generated by inserting tTA-FNF into the Not I– Asc I site of the pGP109(NA). WT and mutant Grp alleles were detected using: GRP forward, 5′-GGACAACGCACTCTCAGCCTAGT-3′; GRP WT reverse: 5′-GAGACGGGGCTCCCTCTAGCTAG-3′; and GRPtTA reverse: 5′-AGTCGACCTTGCGCTTCTTCTT-3′. Generation of the tetO-Stat4A:GFP transgenic mice. The human Stathmin4A cDNA (gift from Andre Sobel) was fused with green fluorescent protein (GFP) cDNA and inserted into pMM400 (gift from Mark Mayford). Genotyping was performed with tetO forward: 5′-GGTCCAACTGCAGCCCAAGC-3′; WT FW4838: 5′-AGCCTAGCTGTTCTCAGCCCCA-3′; WT reverse: 5′-GGGTCTTTGGATTCTTTGTTCTTCCG-3′. Stat4A mice. WT and double-mutant mice were generated by breeding GRP tTA with tetO-Stat4A:GFP mice. Stathmin −/− mice were maintained on C57BL/6J background ( N >10). All mice were maintained on a 12-h light/dark cycle in groups of four to five per cage. Behavioural experiments were conducted during the light phase of the cycle. Mice were 2–4 months (for young adult), 12 months (for middle-aged) or 16–20 months old (for aged) at the time of the experiments. This study was carried out in a strict accordance with the recommendations in the Guide for the Care and Use of Laboratory Animals of the National Institutes of Health. The Rutgers University Institutional Animal Care and Use Committee approved the protocol. Contextual fear conditioning For single foot-shock contextual fear conditioning [17] , on the training day, a mouse was placed in the conditioning chamber (Med Associates) for 148 s before the onset of 2 s of the foot shock (0.75 mA). After an additional 30 s in the chamber, the mouse was returned to its home cage. Thirty minutes or 24 h after training, freezing was assessed for 3 min by FreezeView software (Coulbourn Instrument). For three foot-shock contextual fear conditioning, the mouse was placed in the conditioning chamber for 300 s during which the mouse received three foot shock (0.75 mA, 2 s) with the intertrial interval (ITI) around 58 s. Before the onset of the first US, the mouse was allowed to explore the box for 148 s. After the last US, the mouse stayed in the box additional 30 s before returning to its home cage. Testing was carried out 24 h later, as described above. Cued fear conditioning For single-shock cued fear conditioning [62] , on the training day, a mouse was placed in the conditioning chamber for 2 min before the onset of the conditioned stimulus (CS), a tone that lasted for 30 s at 2,800 Hz, 85 dB. The last 2 s of the CS was paired with the US, 0.75 mA of continuous foot shock. After additional 30 s in the chamber, the mouse was returned to the home cage. Twenty-four hours after the training, mice were placed in an unfamiliar chamber in which the tone (120 s) that had been presented during training was given after a 1-min habituation period (pre-CS). The freezing response was assessed as described above. Morris water maze The task was composed of three training phases [63] , [64] . The first phase consisted of 2 days of training a mouse to reach a visible platform followed by the second phase consisting of 4 days of training to find a hidden platform. A probe trial was performed on the fifth day, 24 h before starting the third phase consisting of a transfer task with a hidden platform located in the quadrant opposite to the location of the platform during the spatial phase. For each phase, four trials, 90 s maximum with a 15-min ITI, were given daily. If the mouse found the platform, it was allowed to rest on it for 20 s before being removed from the pool and placed back into its home cage. If the mouse did not locate the platform within 90 s, the animal was hand guided to it. The animals’ trajectories were recorded with a video tracking system (HVS Image Analyzing VP-118). Appetitive barnes maze A modified version of the original task [65] was used in which a mouse had to find the recessed chamber under one of the holes (target box) to receive food. A circular paltform (90 cm) with 40 holes (hole diameter 5 cm) along the perimeter was used. Mice learned the spatial location of the target box during 4 days of training. Four trials of 300 s maximum with a 30-min ITI interval were given daily. If the mouse found the target box, five pellets (millet seeds) were given inside the target box. If a mouse did not find the platform within 300 s, the animal was hand guided to it and five pellets were given. For this task, the food ration was adjusted individually for the mice to reach 82% of their ad libitum weights. Open-field test The open field [62] consisted of a white arena (43.2 cm × 43.2 cm × 40 cm) coupled to an automated video tracking system (Open Field Activity Software, Med Associates). A mouse was placed in the periphery of the arena and the time spent in the centre of the arena and the total path length were measured. Results were expressed as the per cent of the time spent in the centre over the total time spent in the arena. Elevated plus maze The elevated plus maze [62] (1 m above the floor) consisted of a centre platform (10 cm × 10 cm), two open arms (40 cm × 10 cm) and two closed arms (40 cm × 10 cm) within walls (height 30 cm). A mouse was placed in the centre of the apparatus and the time spent in each arm was measured for 5 min using Limelight software (Coulbourn Instruments). Results were expressed as the per cent of the time spent in open arms over the total time spent in the maze. Forced swim test A mouse was placed [66] in the water tank (24 cm high × 19 cm in diameter filled with 23–25 °C water to a depth of 15 cm) for 5 min, and the total duration of immobility (that is, the time during which the animal made only the small movements necessary to keep its head above water) was measured. Sucrose preference test A mouse was habituated to drink water from two bottles for 7 days [67] . Next, it was subjected to 48 h of forced exposure to 1% sucrose solution to avoid neophobia. Mice were subjected to water deprivation for 16 h before the sucrose preference test was performed. Two pre-weighed bottles, one containing tap water and the other containing 1% sucrose solution, were presented to each animal for 4 h. The position of the water and sucrose bottles (left or right) was switched every 2 h. The bottles were weighed again, and the weight difference represented the animal’s intake from each bottle. The sum of water plus sucrose intake was defined as the total intake, and sucrose preference was expressed as the percentage of sucrose intake relative to the total intake. Immunohistochemistry Mice were anaesthetized with avertin (250 mg kg −1 intraperitoneally) and perfused with 4% paraformaldehyde in 1 × PBS. Their brains were post fixed overnight in 4% paraformaldehyde and cryoprotected in 30% sucrose in 1 × PBS. The brains were sectioned (30 μm) using a cryostat, and single or double labelling immunohistochemistry was performed. Primary antibodies included the mouse monoclonal antibodies against NeuN (1:1,000, Millipore) and glial fibrillary acidic protein (1:500, Millipore), and the rabbit polyclonal antibodies against GFP (1:500, Invitrogen) and adenylate cyclase III (1:100, Santa Cruz). Secondary antibodies were conjugated with Alexa Fluor 488 or 568 (1:500, Molecular Probes) or Cy3 (Jackson ImmunoResearch). Images were acquired using an LSM 510 META laser confocal microscope (Zeiss). Subcellular fractionation The dentate gyrus was isolated [68] and for whole tissue lysates, freshly dissected tissues were homogenized in ice-cold RIPA buffer (50 mM Tris, pH 8.0, 1% TritonX-100, 0.1% SDS, 150 mM NaCl) containing protease and phosphatase inhibitor cocktail tablets (Roche Applied Science). Synaptosomal, PSD and non-PSD fractions were isolated using protocol [17] , [30] , [31] with minor modifications. In brief, pooled dissected tissues from the dentate gyri of three to four mice were homogenized in cold buffer containing 0.32 M sucrose, 50 mM sodium fluoride and 10 mM HEPES, pH 7.4. Homogenates were cleared two times at 1,000 g for 10 min to yield the nuclear enriched pellet and the S1 fraction. To obtain S2 fraction, the S1 fraction was centrifuged and the supernatants (microsomes and cytosol) were collected. To obtain the synaptosomal fraction, the S1 fraction was passed through a nitrocellulose filter (5 μm, Millipore) and spun at 1,000 g for 20 min. The synaptosomal pellet was rinsed twice (4 mM HEPES, 1 mM EDTA, pH7.4, 20 min at 12,000 g ). The resulting pellet was incubated in 20 mM HEPES, 100 mM NaCl, 0.5% Triton X-100, pH7.2, for 15 min and centrifuged. The supernatant (triton-soluble NP fraction) containing non-PSD membranes was retained. The pellet was resuspended in buffer containing 20 mM HEPES, 0.15 mM NaCl, 1% Triton X-100, 1% deoxycholic acid, 1% SDS, pH 7.5, for 1 h and centrifuged at 10,000 g for 15 min. The supernatant contained the PSD or Triton-insoluble fraction. Nuclear fraction was isolated as previously reported [30] , the nuclear-enriched pellets were solubilized in 200 μl nuclear buffer containing 10 mM HEPES/KOH, 10 mM KCl, 10 mM EDTA, 1.5 mM MgCl2, 0.2% BSA, 1 mM dithiothreitol, 0.4% NP40, protease and phosphatase inhibitors, followed by gentle rotating. Samples are centrifuged and the pellets retained as the crude nucleus fraction. Pellets were washed with 500 μl nuclear buffer, followed by centrifugation. Pellets were solubilized (20 mM HEPES/KOH, 400 mM NaCl, 1 mM EDTA, 10% glycerol, 1 mM dithiothreitol, protease and phosphatase inhibitors) followed by gentle vortexing. Samples were gently rotated, vortexed (3 s) and centrifuged to yield the nuclear extract (supernatant) and the nuclear envelope (pellet). Microtubule fractionation was performed as previously reported [17] . In brief, the pooled dissected tissues from the dentate gyrus of three to four mice were homogenized in 400 μl of microtubule stabilizing buffer MTSB (0.1 M PIPES, pH 6.9, 2 M glycerol, 5 mM MgCl 2 , 2 mM EGTA, 0.5% Triton X-100, 4 μg ml −1 Paclitaxel, 5 μg ml −1 pefabloc SC, 5 μg ml −1 leupeptin) and ultracentrifuged at 32,000 g for 20 min at 4 °C. The resulting pellet was resuspended in the MTSB buffer. All buffers were supplemented with protease and phosphatase inhibitors (Roche Applied Science). Protein concentration was measured by BCA protein assay (Thermo Scientific). Western blotting Western blotting was performed [67] , [69] with equal amount of proteins separated on 7% or 12% Bis-Tris gels (Life Technologies) and transblotted onto polyvinylidene difluoride membranes (GE Healthcare Bio-Sciences). Antibodies were against stathmin (1:5,000; kindly provided by Dr A. Sobel), phospho-stathmin (S16, S25, S38) (1:1,000, kindly provided by Dr A. Sobel), tyrosinated tubulin (1:2,000, Sigma), detyrosinated-tubulin (1:5,000, Millipore), α-tubulin (1:5,000, Sigma), β-actin (1:5,000, Sigma), glyceraldehyde 3-phosphate dehydrogenase (1:5,000, Millipore), GM130 (1:2,000, Sigma), Histone H4 (1:2,000, Abcam), SNAP25 (1:2,000, Sternberger Monoclonals), Neuroligin1 (1:1,000, Synaptic Systems), synaptophysin (1:4,000, Sigma), GFP (1:1,000, Life Technologies), GluA2 (1:500, Millipore), KIF5 (1:2,000, Millipore), GluN1 (1:500, Millipore), GluN2A (1:500, Millipore), GluN2B (1:500, Millipore), or PSD95 (1:1,000, Millipore). After incubation with appropriate horseradish peroxidase (HRP)-conjugated secondary antibodies (HRP-linked anti-mouse IgG or HRP-linked anti-rabbit IgG antibody, Cell Signaling), the blots were developed using the ECL-Plus detection Kit (GE Healthcare Bio-Sciences or Thermo Scientific). When the phospho-specific antibodies were used, all buffers included sodium fluoride (50 mM). Densitometric analysis was performed by ImageQuant software (GE Healthcare) after scanning (Typhoon, GE Healthcare). Each experiment was independently repeated at least two times. Full scans of all western blots are provided in Supplementary Figs 14 and 15 . Immunoprecipitation Immunoprecipitation was performed [67] using the synaptosomal fraction from the pooled dissected tissues from the dentate gyrus of four to five mice (for Fig. 1b and Supplementary Fig. 4 ) or pooled whole cell lysate from the hippocampus of two to three mice (for Fig. 8a–c ) were used for the immunoprecipitation experiments. The lysates (1–2 mg of protein) were precleared with Protein G Plus Agarose beads (Thermo Scientific) and with 2–5 μg of anti-α-tubulin (Sigma), anti-KIF5 (Millipore), or normal mouse IgG antibodies (Santa Cruz Biotechnology), followed by incubation with Protein G Plus Agarose beads. The beads were washed five times with RIPA buffer. Proteins were eluted with a sample buffer containing 1% SDS. Western blot analyses of the immunoprecipitated anti-α-tubulin, anti-KIF5, and normal mouse IgG samples and the input (from the precleared step) samples were performed with anti-stathmin, anti-GluA2, anti-KIF5, anti-α-tubulin, or anti-actin antibodies as described above. HRP-conjugated horse anti-mouse IgG antibody (Cell Signaling), HRP-conjugated goat anti-rabbit IgG antibody (Cell Signaling), or HRP-conjugated goat anti-mouse IgG light-chain specific antibody (Jackson ImmunoResearch) were used as secondary antibody. Surgery Mice were anaesthetized with avertin (250 mg kg −1 ) and stainless steel guide cannulae (28 gauge, Plastics One) were implanted into the hippocampus (−2.0 mm anteroposterior (AP), ±1.5 mm mediolateral (ML), −2.0 mm dorsoventral (DV) [70] ). Seven days after surgery, mice were subjected to the experiments. For drug infusion of C57BL/6J mice injected with AAV ( Fig. 8f ), we carried out two surgeries: first, we injected the AAV-GFP or AAV-Stat4A-IRES-GFP (see ‘AAV work’), then performed cannula surgery at least 2 weeks after the AAV virus was expressed. Drug and peptide injection Paclitaxel and nocodazole (Sigma) were used in 5% hydroxypropyl β-cyclodextrin vehicle (wt/vol), at concentrations 10 and 30 nM, respectively. Drugs were fused (0.5 μl per hemisphere) through the cannula at a rate 0.1 μl min −1 . At the end of experiments, we confirmed the injection site by injecting 0.5 μl of methylene blue solution bilaterally, followed by histological analysis of coronal brain slices. Mice that did not receive symmetrical and bilateral injections in the dentate gyrus region of the dorsal hippocampus were excluded from the study. Doxycycline (dox, 40 mg kg −1 , Bio-Serv) was given to mice (2 months of age) for 3 weeks to fully repress the transgene expression. TAT-GluA2 3Y (TAT- 869 YKEGYNVYG 877 ) [34] or TAT-only control peptides (GenScript) at 15 pmol per side in a volume of 0.5 μl saline were bilaterally infused into the dorsal hippocampus. Surgery and cannulae implantation were done as described above. Cannula placement was verified histologically and only mice with adequate cannula replacement were included in subsequent data analysis. AAV work AAV-mediated gene transfer was performed [66] , [67] using plasmid DNAs pAAV-MCS (cytomegalovirus promoter, Stratagene) carrying Stat4A-IRES-GFP or GFP cDNA. AAV viruses (serotype 2) were generated and purified in Vector Biolabs. The genomic titre of each virus was determined using real-time PCR. For virus injections, mice were anaesthetized intraperitoneally with avertin (250 mg kg −1 ) and placed in a stereotaxic frame. The skull was exposed and a small portion of the skull over dorsal hippocampus was removed bilaterally with a drill. Subsequently, AAV vectors (1.0 × 10 12 viral genomes per ml) dissolved in physiological saline were injected bilaterally into the dorsal dentate gyrus (AP: −2.0 mm, ML: ±1.2 mm, DV: −2.0 mm (0.25 μl volume) and −2.4 mm (0.25 μl volume) from the bregma [70] ) at a rate of 0.l μl min −1 . The needle was slowly withdrawn after 3 min. Mice were allowed to recover for 3 weeks after surgery and then subjected to fear conditioning. Successful transduction of the dentate gyrus region was confirmed histologically by immunohistochemistry with GFP. Only mice with strong bilateral GFP expression in target region were included in subsequent data analysis. Electrophysiology Hippocampal slice preparation . Transverse hippocampal slices (400 μm) were obtained from adult (2–3 months old) Stat4A and WT littermate mice. All procedures were performed in compliance with the Institutional Animal Care and Use Committee of the State University of New York, Downstate Medical Center. Slices were cut in ice-cold artificial cerebrospinal fluid (ACSF containing: (in mM) 119 NaCl, 4.0 KCl, 1.5 MgSO 4 , 2 .5 CaCl 2 , 26.2 NaHCO 3 , 1 NaH 2 PO 4 and 11 glucose saturated with 95% O 2 , 5% CO 2 ) and then warmed in oxygenated ACSF to 35 °C for 45 min. Slices were thereafter allowed to equilibrate for at least 60 min in oxygenated ACSF at room temperature. For experiments, slices were immersed in a submerged recording chamber subfused with oxygenated ACSF at 35–36 °C. Field recordings . Field excitatory postsynaptic potentials from the dentate gyrus area were obtained via stimulation with bipolar electrodes (FHC & Co, ME, USA) and recording with borosilicate glass pipettes (5–10 mΩ) filled with ACSF solution. Responses from perforant pathway to granule cell synapses were obtained with a pair of stimulation and recording electrodes located in the dentate gyrus stratum moleculare. For activation of the Schaffer collateral to CA1 synaptic input, stimulation and recording electrodes were placed in the stratum radiatum of the CA1 area. Test pulse intensity was set at ~40% of the maximum field excitatory postsynaptic potential slope. Test sampling was 0.017 Hz (once per minute) and test pulse duration was 50 μs. LTP was induced by θ -burst stimulation: three bursts spaced by 20 s, each burst consisting of 6 trains of high-frequency stimulus (6 pulses at 100 Hz) delivered at 10 Hz. Statistical analysis Differences in protein expression between groups were determined using one-way ANOVA or two-way ANOVA, with Fisher’s LSD post-hoc tests. The behavioural data were examined using a Student’s t -test, one-way ANOVA or two-way ANOVA with Bonferroni correction. The electrophysiological data were analysed with two-way repeated measure ANOVA. In all cases, P- values were two-tailed and the comparisons were considered statistically significant when P <0.05. All data are presented as the mean±s.e.m. How to cite this article: Uchida, S. et al. Learning-induced and stathmin-dependent changes in microtubule stability are critical for memory and disrupted in ageing. Nat. Commun. 5:4389 doi: 10.1038/ncomms5389 (2014).